Fracture toughness of graphene Perfect graphene is believed to be the strongest material. However, the useful strength of large-area graphene with engineering relevance is usually determined by its fracture toughness, rather than the intrinsic strength that governs a uniform breaking of atomic bonds in perfect graphene. To date, the fracture toughness of graphene has not been measured. Here we report an in situ tensile testing of suspended graphene using a nanomechanical device in a scanning electron microscope. During tensile loading, the pre-cracked graphene sample fractures in a brittle manner with sharp edges, at a breaking stress substantially lower than the intrinsic strength of graphene. Our combined experiment and modelling verify the applicability of the classic Griffith theory of brittle fracture to graphene. The fracture toughness of graphene is measured as the critical stress intensity factor of and the equivalent critical strain energy release rate of 15.9 J m −2 . Our work quantifies the essential fracture properties of graphene and provides mechanistic insights into the mechanical failure of graphene. Graphene [1] is a promising candidate in a number of electrical, thermal and mechanical applications, owing to its exceptional physical properties [2] , [3] , [4] . Graphene also attracts great attention as the strengthening component in composites [5] , [6] , [7] . Characterization of the mechanical properties of graphene is essential both from a technological perspective for its reliable applications and from a fundamental interest in understanding its deformation physics [8] , [9] . In materials science, fracture toughness is a property that describes the ability of a material containing a crack to resist fracture, and is one of the most important mechanical properties of any material [10] , [11] . The useful strength of large-area graphene with engineering relevance is usually determined by its fracture toughness, rather than the intrinsic strength that dictates a uniform rupture of carbon bonds in graphene. Theoretical and computational modelling in recent literature has provided important insights into the fracture and strength-controlling mechanisms of graphene with both perfect and defective lattice structures [12] , [13] , [14] , [15] , [16] , [17] , [18] , [19] , [20] , [21] , [22] . However, the fracture toughness of graphene has not been experimentally measured to date. Graphene has an extremely small dimension in thickness, on the order of the nanometre scale. It has been a challenge to quantitatively measure the mechanical properties of graphene, owing to technical difficulties in the nanomechanical testing of atomically thin membranes. The pioneering mechanical testing of graphene has been conducted by Lee et al. [23] through nanoindentation of freely suspended graphene films in an atomic force microscope. They reported Young’s modulus and intrinsic strength of the mechanically exfoliated pristine graphene as 1 TPa and 130 GPa, respectively. The comparable elastic stiffness and intrinsic strength were also measured for chemical vapour deposition (CVD) synthesized polycrystalline graphene [24] . On the other hand, the morphologies of fractured graphene have been studied qualitatively by the optical and scanning electron microscopy (SEM) observation of the graphene films on substrates, as well as by the transmission electron microscopy (TEM) imaging of fracture edges of suspended graphene membranes [19] , [25] . Whereas these experimental fracture studies provide ‘visible’ results, methods used are neither easily controllable nor straightforward, which underscores the critical need of development of a direct and quantitative approach to test the fracture properties of graphene. Here we report the quantitative in situ nanomechanical testing of the fracture toughness in CVD-synthesized graphene. Brittle fracture was observed in the freestanding graphene films containing a central crack, which was introduced by focused iron beam (FIB) cutting. The critical tensile stresses of fracture were measured for different initial crack lengths. These data enable us to verify the applicability of the classic Griffith theory [10] , [11] to the brittle fracture of graphene. From these data, we further determine the fracture toughness of graphene measured by the critical stress intensity factor, as well as the critical strain energy release rate of fracture. Our molecular dynamics (MD) simulations provide validation and insight for experimental results. This work represents the first measurement of the fracture toughness of graphene. Broadly, it provides an effective strategy of the nanomechanical testing of fracture properties for emerging two-dimensional (2D) materials [26] . Dry transfer of graphene A critical step in the nanomechanical testing of graphene was to transfer the atomically thin film of as-grown graphene onto a sample stage. To this end, we developed a unique approach of dry transfer. Here, the ‘dry’ transfer is emphasized because liquid is unfavourable for the suspended Si working layer of the stage. Specifically, graphene was synthesized by CVD on a copper foil. The as-grown graphene was first coated by poly (methyl methacrylate) (PMMA) and then attached to a polydimethylsiloxane (PDMS) block. The PDMS block has an open window slightly larger than the sample stage in the center and can attach to graphene/PMMA by natural adhesion ( Fig. 1a,b ). The PDMS/PMMA/graphene block was easily picked up from the etchant after copper was etched away in several hours, so that it was transferred directly onto the stage ( Fig. 1c ). The whole stage was then covered by the PMMA/graphene film in the central window of the PDMS block. Heat treatment enabled the PMMA/graphene film to adhere to the suspended Si layer of the device smoothly and tightly, which was important to prevent wrinkle formation and release pre-strain in the graphene film. Afterwards, the graphene/PMMA film was carefully cut with a sharp tip of tweezers along the open window contour of the PDMS block, and the sample stage together with the transparent graphene/PMMA film was subsequently picked up with tweezers ( Fig. 1d,e ). After calcining in air to decompose PMMA, a suspended film of graphene was obtained across the stage ( Fig. 1f ). 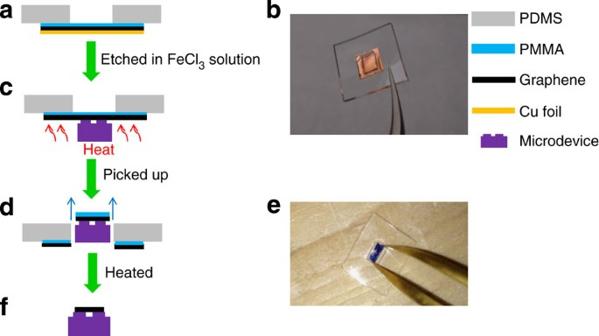Figure 1: Schematic illustration of the dry transfer method. (a–f) Sequential steps of dry transfer. The two blue arrows in (d) show the position where the device was picked up together with graphene/PMMA by tweezers. (b,e) correspond to schematic (a,d), respectively. Figure 1: Schematic illustration of the dry transfer method. ( a – f ) Sequential steps of dry transfer. The two blue arrows in ( d ) show the position where the device was picked up together with graphene/PMMA by tweezers. ( b , e ) correspond to schematic ( a , d ), respectively. Full size image Characterization of graphene morphology Both SEM and TEM were used to characterize the morphology of suspended graphene on the sample stage. To prepare samples for in situ tensile testing, the suspended graphene with a relatively flat and clean surface was selected through SEM observation ( Fig. 2a ), and then cut into the rectangular shape by FIB. TEM images of the suspended graphene show discontinuous PMMA residues ( Fig. 2b ). It is difficult to entirely avoid PMMA residues even for the more established transfer method with acetone as solvent. PMMA is, however, well known as a soft polymer, which is not supposed to have a significant influence on the mechanical properties of strong and brittle graphene. Diffraction patterns (inset in Fig. 2b ) demonstrate the high quality of graphene, in spite of some rings from polymer residues. Samples are polycrystalline with grain sizes in the range of hundreds of nanometres to a few microns. They are primarily bilayer graphene as shown in the TEM images of graphene edges, though the monolayer one is occasionally observed ( Fig. 2c,d ). The structure of bilayer graphene is further confirmed by Raman spectra, as shown in the insets of Fig. 2c,d . The ratio of 2D/G intensity is used to evaluate the thickness of graphene, especially for few-layered graphene: its value is ~1 for bilayer graphene and >3 for monolayer graphene, as discussed in previous studies [27] . The spacing between graphene layers is estimated to be about 0.34 nm (ref. 28 ). 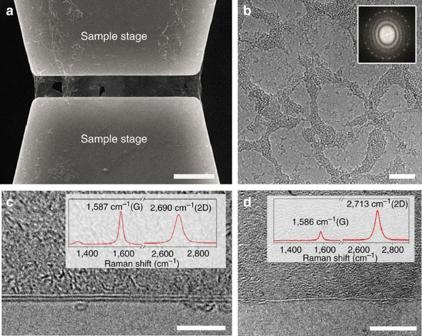Figure 2: Characterization of the suspended graphene sample. (a) SEM image showing a suspended graphene film prepared by the dry transfer method (scale bar, 5 μm). (b) TEM image showing the morphology of a suspended graphene sample with discontinuous polymer residue (scale bar, 10 nm). Inset inbis the corresponding fast Fourier transform diffraction pattern of this polycrystalline graphene. (c,d) TEM and Raman characterizations confirm the sample structure on the edges. For the bilayer and monolayer graphene, the ratio of 2D/G is ~1 and >3, respectively (scale bar, 5 nm (c), scale bar, 10 nm (d)). Figure 2: Characterization of the suspended graphene sample. ( a ) SEM image showing a suspended graphene film prepared by the dry transfer method (scale bar, 5 μm). ( b ) TEM image showing the morphology of a suspended graphene sample with discontinuous polymer residue (scale bar, 10 nm). Inset in b is the corresponding fast Fourier transform diffraction pattern of this polycrystalline graphene. ( c , d ) TEM and Raman characterizations confirm the sample structure on the edges. For the bilayer and monolayer graphene, the ratio of 2D/G is ~1 and >3, respectively (scale bar, 5 nm ( c ), scale bar, 10 nm ( d )). Full size image In situ tensile testing Quantitative in situ tensile testing was performed using a recently developed platform that integrates a micromechanical device [29] and a nanoindenter [30] , [31] , [32] , as shown in Fig. 3a . A central pre-crack with length <10% of sample width ( Fig. 3b ) was introduced by FIB. The tensile testing was closely monitored by real-time SEM observation. As the applied load was increased to a critical value, brittle fracture occurred quickly from the pre-crack, resulting in two fractured pieces with flat edges. 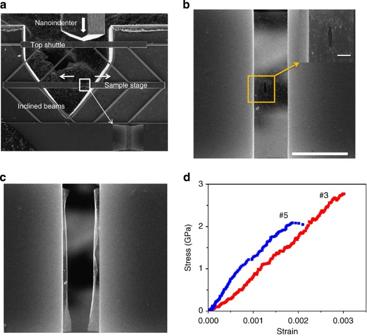Figure 3: Nanomechanical testing of fracture of graphene with a pre-crack. (a) SEM image showing thein situtensile testing with a microdevice. Movement of the nanoindenter tip (shown by the block arrow) was converted to pure tension of the specimen on the sample stage by the inclined beams. Inset is the magnified image of the boxed region showing graphene across the gap of the sample stage. (b,c) SEM images showing graphene on the sample stage before and after tensile testing, respectively. The pre-crack (boxed in (b)) was cut by FIB. The scale bar in (b) and its inset is 5 μm and 500 nm, respectively. (d) Selected engineering stress-strain curves of the cracked graphene samples (corresponding to #3 and #5 inTable 1). Figure 3b,c shows the SEM snapshot of graphene before and after fracture, respectively. But we were not able to use SEM to record a clear process of fast crack growth. The brittle fracture is also manifested in the linear stress-strain curve ( Fig. 3d ), which ends by an abrupt load drop signifying the start of dynamic crack propagation. Table 1 lists the initial crack length 2 a 0 and corresponding fracture stress σ c from the testing of five samples. Owing to the weakening effect of pre-crack, these measured fracture stresses are substantially lower than the intrinsic strength of graphene with an estimated value of ~100 GPa (ref. 33 ), which corresponds to the critical tensile stress of uniform rupture of atomic bonds in pristine graphene. Figure 3: Nanomechanical testing of fracture of graphene with a pre-crack. ( a ) SEM image showing the in situ tensile testing with a microdevice. Movement of the nanoindenter tip (shown by the block arrow) was converted to pure tension of the specimen on the sample stage by the inclined beams. Inset is the magnified image of the boxed region showing graphene across the gap of the sample stage. ( b , c ) SEM images showing graphene on the sample stage before and after tensile testing, respectively. The pre-crack (boxed in ( b )) was cut by FIB. The scale bar in ( b ) and its inset is 5 μm and 500 nm, respectively. ( d ) Selected engineering stress-strain curves of the cracked graphene samples (corresponding to #3 and #5 in Table 1 ). Full size image Table 1 Experimental data of crack size and critical fracture stress for bilayer graphene with a pre-crack of length 2 a 0 . Full size table Griffith’s brittle fracture To understand the above fracture experiments, an important question to address is whether the classic Griffith theory of brittle fracture [9] , [10] is applicable to graphene or not, since it has never been directly tested for 2D materials such as graphene. According to Griffith [10] , brittle fracture occurs when the decrease of strain energy exceeds the increase of surface energy for an infinitesimal extension of the crack. For a central crack of length 2 a 0 , the Griffith criterion expresses the critical stress of onset of fast fracture, σ c , as a function of a 0 , rather than a constant value of the intrinsic stress of bond breaking [10] . In equation (1), E is Young’s modulus and γ is the surface energy (that is, the edge energy for a 2D material like graphene). The Griffith criterion of equation (1) can be rewritten as so that the left-hand side of equation (2) contains only the experimentally measured fracture quantities (that is, fracture stress and crack size), while the right-hand side depends only on the material and numerical constants; such grouping of parameters was originally used by Griffith [10] . According to equation (2), the Griffith theory of brittle fracture is applicable to graphene, if the experimentally measured pairs of σ c and a 0 give a constant product of . As listed in Table 1 , the measured values of range from and are distributed evenly around an average value of , with a standard deviation (s.d.) of . These results indicate that the measured can be approximately considered as a constant, by noting the difficulties and accordingly the uncertainties associated with sample preparation, transfer and quantitative nanomechanical testing of atomically thin membranes. Hence, our experiments provide a direct proof that the Griffith theory of brittle fracture is applicable to graphene. Note that the graphene samples tested are mostly bilayer films. Therefore, a thickness of 0.68 nm for the bilayer graphene is used to convert the measured fracture force to the tensile fracture stress in Table 1 . Because of the brittle nature of graphene, its useful strength with engineering relevance should be dictated by fracture toughness, which is conventionally characterized by the critical stress intensity factor of fracture, . Given the measured values of in Table 1 , we obtain , with a s.d. of for graphene. The fracture toughness is also often given by the critical strain energy release rate of fracture, . With Young’s modulus of graphene E =1 TPa, we obtain the measured value of . According to equation (1), we estimate the edge energy of graphene as γ = G c /2=8.0 J m −2 . To understand the above experimental results, we performed MD simulations of brittle fracture in pre-cracked graphene. The simulated freestanding graphene slab has a smaller size (60 nm in width and 30 nm in height) but a similar aspect ratio as experimental samples. 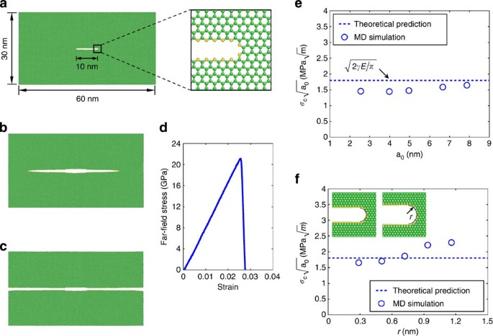Figure 4: Molecular dynamics (MD) simulations of brittle fracture in a monolayer single-crystal graphene with a pre-crack. (a) Atomic structure of a graphene slab containing a central crack. The zoom-in image shows the near-tip structure as well as the crack face with the zigzag edge. (b) An intermediate state of fast crack propagation. (c) The final state of cleavage fracture, resulting in atomically smooth edges. (d) Corresponding stress-strain curve of the pre-cracked graphene during fracture. (e) Effect of the pre-crack length 2a0on the product of. (f) Effect of blunting of the crack tip with different notch radii ofr. In (e,f), MD results (circles) are compared with the prediction (dashed line) from the Griffith theory of brittle fracture. Figure 4a shows the atomic configuration of a monolayer single-crystal graphene containing a central crack of length 2 a 0 , which is introduced by removing a few layers (that is, a short segment in 2D) of carbon atoms, resembling the crack cutting by FIB in experiment. The crack face is taken along the zigzag direction. Periodic boundary conditions are imposed, and the system is free to relax along the horizontal direction. The far-field tensile load, normal to the crack face, is increased incrementally in a strain-controlled manner, and the system temperature is maintained at T =300 K. Figure 4d shows the MD stress-strain curve for a pre-cracked graphene slab that exhibits a nearly linear response, which ends at a sudden load drop corresponding to the brittle facture of fast crack propagation through the entire slab. The brittle fracture is also manifested as the formation of atomically smooth fracture edges as in Fig. 4b,c . As in the experiments, an increase of the initial crack length 2 a 0 leads to a decrease of the fracture stress σ c in MD. Figure 4e shows that the calculated product of is approximately a constant, and it approaches the theoretical prediction of as the initial crack becomes longer, thereby geometrically approaching the ideal Griffith crack that should be long and sharp. Hence MD results corroborate the experiments on the applicability of the Griffith theory to brittle fracture in graphene. The corresponding critical strain energy release rate of fracture G c from MD is 11.8 J m −2 . This result is consistent with a recent atomistic prediction of the fracture toughness of graphene [17] as 3.82 × 10 −9 J m −1 , which corresponds to a bulk value of 11.2 J m −2 , assuming a graphene thickness of 0.34 nm. MD predictions of the Griffith fracture in monolayer graphene are also consistent with those in bilayer graphene ( Supplementary Fig. 1 ; Supplementary Discussion ). This is because the van der Waals interaction between graphene layers is much weaker than the covalent carbon bonding within the graphene layer, such that the interlayer interaction has a negligibly small effect on the in-plane fracture response. Our MD prediction of G c is about 26% lower than the average value of experimental measurements. This discrepancy arises likely owing to the influences of crack blunting, crack orientation, polycrystal microstructure, defect formation, lattice trapping, and so on. Figure 4: Molecular dynamics (MD) simulations of brittle fracture in a monolayer single-crystal graphene with a pre-crack. ( a ) Atomic structure of a graphene slab containing a central crack. The zoom-in image shows the near-tip structure as well as the crack face with the zigzag edge. ( b ) An intermediate state of fast crack propagation. ( c ) The final state of cleavage fracture, resulting in atomically smooth edges. ( d ) Corresponding stress-strain curve of the pre-cracked graphene during fracture. ( e ) Effect of the pre-crack length 2 a 0 on the product of . ( f ) Effect of blunting of the crack tip with different notch radii of r . In ( e , f ), MD results (circles) are compared with the prediction (dashed line) from the Griffith theory of brittle fracture. Full size image MD simulations allow us to directly assess the influence of crack blunting on the measured fracture toughness. As shown in the inset of Fig. 4f , multiple layers of atoms are removed to create the blunt crack tip with a notch radius of r , while keeping the same crack length of 2 a 0 =16 nm. Compared with the atomically sharp crack tip, the blunt notch reduces the local stress concentration within a distance of order r , so that the far-field fracture stress has to increase with r . As shown in Fig. 4f , when r is increased from 0.3 to 1.2 nm (that is, 0.03 to 0.15 a 0 ), (equivalent to K c ) increases by about 30%. Note that the sample sizes in MD simulations are kept much smaller than those in experiments, so as to reduce the computational cost. In addition, the use of different aspect ratios of samples could affect the quantitative outcome of MD results. Nonetheless, the trend of fracture stress increasing with tip radius is captured in Fig. 4f . In the experiment, we were not able to directly visualize the atomic structure of the crack tip for evaluating the effects of crack blunting on the measured fracture toughness, owing to the limitations in the current experimental setup. The crack blunting effect warrants further study in the future. MD simulations are also performed to evaluate the influence of crack orientation on fracture load. Owing to the rotational symmetry of the hexagonal lattice of graphene, one only needs to consider crack orientations in between the two limits of armchair and zigzag edges, which differ by an in-plane rotation of 30°. Our MD simulations based on the reactive empirical bond order (REBO) potential show that the fracture stress is the lowest for the zigzag crack edge, and the largest along the armchair one; it varies monotonically for intermediate orientations between the two limits. These results can be correlated to the orientation dependence of the edge energy, 2 γ , which is the lowest of 11.8 J m −2 for the zigzag edge and the highest of 12.5 J m −2 for the armchair edge as predicted by the REBO potential. Such a trend is opposite to that predicted by ab initio calculations as well as by reactive force field (ReaxFF) calculations [19] . However, the computationally intensive ab initio calculation severely limits the size of the simulated cracked system, and the ReaxFF predicts a stress-strain behaviour that exhibits artifacts of discontinuities in elastic deformation. Hence, we report MD results based on the REBO potential by noting that the variation of predicted fracture stresses due to the crack orientation effect is still relatively small compared with that of experimental values. Incidentally, Girit et al. [34] reported that graphene at the edge seems to be dominated by zigzag structures based on in situ observations with an aberration-corrected transmission electron microscope. This result implies that the zigzag edge is more stable with a lower edge energy. Hence, the combined experimental and modelling study is needed to understand the crack orientation effect on Griffith’s fracture in the future. To investigate the crack-tip interaction with grain boundaries, we performed MD simulations of Griffith’s fracture in pre-cracked polycrystalline graphene. 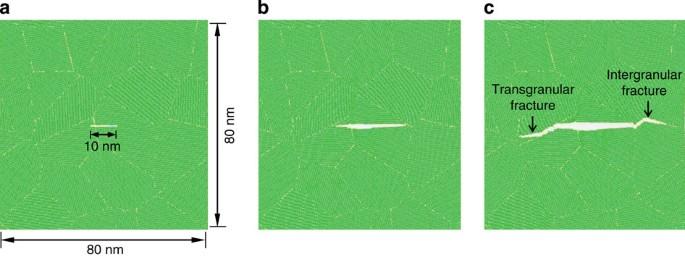Figure 5: Molecular dynamics simulation of brittle fracture in a monolayer polycrystalline graphene with a pre-crack. (a–c) Snapshots of crack growth, exhibiting both intergranular and intragranular fractures. Atoms are coloured by the coordination number (N=3: green; 2: yellow; 4: grey), showing grain boundaries that contain mis-coordinated atoms (N≠3). Figure 5 shows a typical MD result, where both intergranular and intragranular fractures are observed, depending on the crack-tip location as well as the orientation of grain boundary relative to the crack face. Supplementary Figure 2 and Supplementary Discussion show another MD result of Griffith’s fracture in polycrystalline graphene having the same sample geometry as the single-crystal one in Fig. 4a . In this case, the pre-crack length is 10 nm and the simulated fracture stress is 21.1 GPa, giving that approximately satisfies the Griffith criterion of brittle fracture. Incidentally, the intrinsic strength of polycrystalline graphene without a pre-crack might be strongly influenced by the grain boundary characteristics. A recent AFM study of polycrystalline graphene shows that grain boundaries with large mismatch angles can maintain as high as 92% strength of single-crystal graphene, but the presence of low-angle grain boundaries can lower the strength to 59% of that of pristine graphene [35] . In contrast, an earlier publication reported that polycrystalline graphene is almost as strong as pristine samples [24] . While quantifying the intrinsic strength is essential to characterize the fracture properties of graphene without a dominant crack, the present work is focused on fracture toughness as a threshold of initiation of crack growth in graphene with a finite-sized pre-crack. Under these conditions, the influences of grain boundaries on the change of the far-field stress to start crack growth (due to such events as crack deflection or arrest at grain boundaries) are relatively small as shown in Supplementary Fig. 2 . Nonetheless, it is important to further study the effects of interactions between the crack tip and grain boundary on the fracture load in finer detail. Figure 5: Molecular dynamics simulation of brittle fracture in a monolayer polycrystalline graphene with a pre-crack. ( a – c ) Snapshots of crack growth, exhibiting both intergranular and intragranular fractures. Atoms are coloured by the coordination number ( N =3: green; 2: yellow; 4: grey), showing grain boundaries that contain mis-coordinated atoms ( N ≠3). Full size image Finally, we note that the atomic-level processes of breaking of covalent carbon bonds near a crack tip could be accompanied by the defect formation of Stone–Wales pairs that effectively shield the crack and thus increase the required far-field stress to fracture [36] . Moreover, the lattice-trapping effect [16] , [17] , [37] , [38] , which requires an increase of the far-field stress to overcome the energy barriers of crack-tip bond breaking, could also be responsible for the discrepancy between the Griffith stress and the actual fracture stress from the experiment/MD. To summarize, with a successful dry transfer of CVD-synthesized graphene, we conduct the first in situ nanomechanical testing of fracture in suspended graphene with controlled pre-crack sizes. The cracked graphene samples exhibit a fast brittle fracture behaviour with the breaking stress much lower than the intrinsic strength of graphene. Our combined experimental and modelling study provides a direct proof for the applicability of the classic Griffith theory to the brittle fracture of graphene. This result has a significant implication on the useful strength of large-area graphene that should be determined by its fracture toughness, rather than intrinsic strength. Broadly, our work provides an effective approach for the nanomechanical characterization of the fracture properties of emerging 2D materials. We conclude by commenting on the prospect of future research on the strength of graphene. The present quantitative measurement of the fracture toughness of pre-cracked graphene, in conjunction with the early studies of the intrinsic strength of graphene without pre-crack, provides the most essential characterization of the mechanical strength of graphene. In the future, it is also important to investigate the fragility [39] of graphene by studying the ease of formation of a macroscopic crack through the evolution of microcracks under different thermo-mechanical loading conditions. Ultimately, the fragility of a strong solid such as graphene determines its practical utility in engineering applications for advanced devices and composites. Preparation of graphene Graphene was synthesized by CVD on a copper foil with CH 4 as a precursor. The temperature initially rose to 1,000 °C in 15 min in H 2 /Ar and then remained constant during growth. The copper foil was annealed for 20 min before the precursor gas (CH 4 ) was turned on for graphene growth for 8 min at 4 sccm. The whole process was kept under low pressure around 1 torr controlled by a rotary pump. Dry transfer of graphene Copper foil was etched in a FeCl 3 solution before the PDMS/PMMA/graphene block was picked up together. After this block was put on the device, the sample was heated up to 160 °C for 1 h to make PMMA/graphene film attached to the device. Thermal treatment was then employed at a temperature of 320 °C in air for 2 h to remove PMMA. In situ tensile testing Uniaxial tensile testing of graphene was conducted within a FEI Quanta 400 SEM chamber equipped with an InSEM indenter (Agilent Technologies, Oak Ridge, Tennessee) system. The design of the micromechanical device converted the compression from the indenter on the top shuttle to the uniaxial stretch of the sample. Atomistic modelling MD simulations are performed using the large-scale atomic/molecular massively parallel simulator (LAMMPS) [40] . A REBO potential [41] is used to model the interatomic interaction for carbon. Note that the C–C interaction in the REBO potential is prescribed with a switching function, and the original cutoff distances are 1.7 Å and 2.0 Å, respectively. It is known that the switching function with such cutoff distances generates non-physical behaviours under large strains pertinent to fracture, owing to an artifact of high bond forces introduced in the fracture process [42] . To solve this problem, we set the cutoff distances at 1.92 Å, as suggested by previous studies [12] , [13] , [14] , [15] . How to cite this article: Zhang, P. et al. Fracture toughness of graphene. Nat. Commun. 5:3782 doi: 10.1038/ncomms4782 (2014).